Activin induces cortical interneuron identity and differentiation in embryonic stem cell-derived telencephalic neural precursors Understanding the mechanisms underlying neural progenitor differentiation and neuronal fate specification is critical for the use of embryonic stem cells (ESCs) for regenerative medicine. Cortical interneurons are of particular interest for cell transplantation; however, only a limited subset of these neurons can be generated from ESCs. Here we uncover a pivotal role for Activin in regulating the differentiation and identity of telencephalic neural precursors derived from mouse and human ESCs. We show that Activin directly inhibits the mitogenic sonic hedgehog pathway in a Gli3-dependent manner while enhancing retinoic acid signalling, the pro-neurogenic pathway. In addition, we demonstrate that Activin provides telencephalic neural precursors with positional cues that specifically promote the acquisition of a calretinin interneuron fate by controlling the expression of genes that regulate cortical interneuron identity. This work demonstrates a novel means for regulating neuronal differentiation and specification of subtype identity. During neurogenesis, the balance between signalling inputs that control neural progenitor self-renewal and differentiation is critical for the expansion of the stem cell pool or the initiation of the terminal differentiation programme. In the telencephalon, the self-renewal of neural progenitors is thought to be under the tight control of a number of growth factors. For example, sonic hedgehog (Shh), as well as its patterning activities, promotes self-renewal and prevents differentiation within the telencephalon [1] . In contrast to this, retinoic acid (RA) acts as a pro-differentiation factor in a wide variety of neuronal settings [2] , and, in the telencephalon, inhibits progenitor proliferation and promotes neuronal differentiation [3] . How these different growth factor inputs are coordinated to promote self-renewal or differentiation remains unknown. A second key event during neurogenesis is the specification of neuronal subtype identity. The cerebral cortex functions in memory and higher-order cognitive processing. Two classes of neurons carry out these roles, the excitatory glutamatergic projection neurons and the inhibitory GABAergic interneurons. Interneurons, comprising 20–30% of cortical neurons, modulate cortical output [4] and, during corticogenesis, regulate neural progenitor proliferation and migration [5] , as well as postnatal development of the cortical circuitry [6] . Most cortical interneurons can be subdivided into three main subtypes that express parvalbumin, somatostatin or calretinin, and mainly originate from distinct domains within the ventral telencephalon and then migrate to the cortical region [7] . Somatostatin and parvalbumin-type interneurons are specified in the medial ganglionic eminence (MGE) by Shh-mediated induction of Nkx2.1 [8] . In contrast to this, calretinin interneurons form in the caudal ganglionic eminence (CGE) [9] , and the signals that control their specification have not been identified. The ' in vitro ' differentiation of embryonic stem cells provides a powerful tool to understand telencephalic development and is a potential source of cells for use in regenerative medicine. Special attention has been paid to cortical interneurons owing to their remarkable migratory capacity in postnatal cortex, their stereotypic differentiation after transplantation and their regulation of cortical activity [10] , [11] , [12] , [13] . The serum-free monolayer differentiation protocol allows to obtain in a reproducible manner relatively pure populations of telencephalic neural progenitor cells that respond to Shh signalling in the same way as occurs during normal development [14] , [15] . Here, using embryonic stem cell (ESC)-derived neural precursors to identify novel morphogens that pattern the telencephalon, we have found that Activin is a potent neurotrophic factor that induces differentiation into postmitotic neurons. We find that Activin does this in two ways, by promoting cell cycle exit via the inhibition of the Shh pathway and by enhancing RA signalling, a key pathway for neuronal terminal differentiation. Furthermore, we show that Activin signalling also confers positional identity to these neural precursors by directing them towards a CGE fate and therefore induces the formation of calretinin cortical interneurons. Activin induces neural precursor differentiation Activin belongs to the TGFβ superfamily. During telencephalic development, Activin subunits, TGFβs and their receptors are widely expressed [16] and high levels of Smad2/3 activation are observed in the lateral ganglionic eminence (LGE) and CGE [17] . However, very little is known about the roles of this signalling pathway in telencephalic development. To explore the role of Activin signalling, we differentiated mouse ESCs as a monolayer in serum-free media for 5 days [15] , the time point when the highest proportion of neural precursors are present, the expression of pluripotency markers is extinguished and there is a dramatic increase in the expression of ventral telencephalic markers ( Supplementary Fig. S1 ). At this stage, cells were replated into poly- D -lysine- and laminin-coated dishes. This time point was considered as day 0 of our experiments. Day 0 cultures were treated with 10 ng ml −1 of Activin. After 4 days, we observed that Activin-treated cells showed clear morphological signs of differentiation ( Fig. 1a ), reduced rosette formation, a dramatic decrease in the percentage of Nestin + neural precursors and a comparable increase in the proportion of ßβ-III-tubulin + postmitotic neurons ( Fig. 1a ). Activin treatment did not alter the proportion of AnnexinV + or Caspase3 + neural precursors or neurons, indicating that these changes were not due to a pro-survival role of Activin ( Fig. 1b ). Interestingly, TGFβ1 and TGFβ3 did not affect the proportions of neural precursors and neurons of our cultures ( Supplementary Fig. S2 ), indicating that our observations are specific to the Activin members of the TGFβ family. Together, these findings suggested that Activin induces differentiation of telencephalic progenitors into postmitotic neurons. 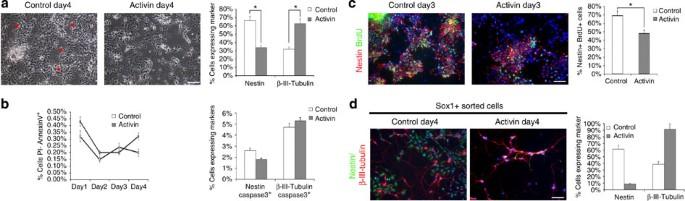Figure 1: Activin induces the differentiation of telencephalic neuronal precursors. (a) Control and Activin-treated cultures illustrating how Activin promotes neural precursor differentiation (arrowheads mark rosettes present in control cultures). The right panel contains a plot of the proportion of Nestin+cells/β-III-tubulin+cells in these cultures: Activin treated 36±5.5/62±9.25% and control treated 62±11.23/35±6.46%. (b) Plot on the left shows the relative number of Annexin V+/PI−vecells in control and Activin-treated cultures (these oscillate between 0.2–0.45% for Activin cultures and 0.15–0.32% for control cultures). The panel on the right displays the Caspase3-positive neural precursors ands neurons in control and Activin-treated cultures. At day 3, 5.3±0.3% of cells in Activin-treated cultures and 4.7±0.3% in control cultures were double Caspase3/β-III-tubulin+and 1.8±0.1% in Activin cultures and 2.6±0.2% in control cultures were double Caspase3/Nestin+cells. (c) Immunofluorescent analysis and quantification of Nestin+/BrdU+cells in control (69±5.2%) and Activin (48±3.84%) cultures after 3 days of treatment showing how Activin-treated precursors proliferate slowly. (d) Sorted Sox1+cells differentiate in response to Activin (Nestin+/β-III-tubulin+cells: Activin cultures 8.69±1.65/91.3±17% and control cultures 61.27±6.32/38.7±4.64%). For all experiments,n=3, mean±s.e.m. Student'st-test. *P<0.001. ESCs were differentiated for 5 days as a monolayer, then replated into poly-D-lysine/laminin-coated dishes and cultured in NBB27 media (controls) or NBB27+10 ng ml−1Activin. For (d), Sox+cells were sorted at day 5 of monolayer differentiation and replated as above. Scale bar=50 μm (aandc) and 25 μm (d). Figure 1: Activin induces the differentiation of telencephalic neuronal precursors. ( a ) Control and Activin-treated cultures illustrating how Activin promotes neural precursor differentiation (arrowheads mark rosettes present in control cultures). The right panel contains a plot of the proportion of Nestin + cells/β-III-tubulin + cells in these cultures: Activin treated 36±5.5/62±9.25% and control treated 62±11.23/35±6.46%. ( b ) Plot on the left shows the relative number of Annexin V + /PI −ve cells in control and Activin-treated cultures (these oscillate between 0.2–0.45% for Activin cultures and 0.15–0.32% for control cultures). The panel on the right displays the Caspase3-positive neural precursors ands neurons in control and Activin-treated cultures. At day 3, 5.3±0.3% of cells in Activin-treated cultures and 4.7±0.3% in control cultures were double Caspase3/β-III-tubulin + and 1.8±0.1% in Activin cultures and 2.6±0.2% in control cultures were double Caspase3/Nestin + cells. ( c ) Immunofluorescent analysis and quantification of Nestin + /BrdU + cells in control (69±5.2%) and Activin (48±3.84%) cultures after 3 days of treatment showing how Activin-treated precursors proliferate slowly. ( d ) Sorted Sox1 + cells differentiate in response to Activin (Nestin + /β-III-tubulin + cells: Activin cultures 8.69±1.65/91.3±17% and control cultures 61.27±6.32/38.7±4.64%). For all experiments, n =3, mean±s.e.m. Student's t -test. * P <0.001. ESCs were differentiated for 5 days as a monolayer, then replated into poly- D -lysine/laminin-coated dishes and cultured in NBB27 media (controls) or NBB27+10 ng ml −1 Activin. For ( d ), Sox + cells were sorted at day 5 of monolayer differentiation and replated as above. Scale bar=50 μm ( a and c ) and 25 μm ( d ). Full size image To test how Activin affects the cell cycle of neuronal precursors, we measured the percentage of Nestin + cells that incorporate BrdU after a pulse of 6 h. When compared with controls, Activin-treated cells showed a significantly lower proportion of neuronal precursors incorporating BrdU ( Fig. 1c ), suggesting that Activin treatment was causing a decrease in the number of neural progenitors re-entering the cell cycle and therefore initiating the differentiation process. The observation that Activin induces differentiation of cultures predominately composed of neural precursor cells ( Supplementary Fig. S1a ) suggests that it is directly acting on this cell type. To confirm this finding, Sox1–green fluorescent protein (GFP) cells [15] were sorted for GFP expression and treated with Activin for 4 days. When this was done, we observed that Activin dramatically decreased the proportion of Nestin + neural precursors and increased the proportion of βß-III-tubulin neurons ( Fig. 1d ). Therefore, we conclude that Activin induces the differentiation of Sox1-expressing telencephalic neural precursor cells into postmitotic neurons. Activin-generated neurons are electrophysiologically active We next investigated the electrophysiological properties of Activin-treated and control cells at day 5 in vitro . Cells were visually identified as neurons and targeted for whole-cell current-clamp recordings ( Fig. 2a ). We observed no differences in resting membrane potential, input resistance or whole-cell capacitance between Activin-treated and control cells (−30.4±14.8 versus −38.9±14.7 mV; 1.9±1.6 versus 1.5±1.3 GΩ; 6.5±3.6 versus 6.3±2.1 pF (Activin versus control, mean±s.d. ); P >0.05, t -tests). To examine their ability to fire action potentials (APs), cells were injected with depolarizing current pulses from their resting membrane potential. We found that cells could be distinguished into four functional subgroups, which presumably reflect different stages in their maturation ( Fig. 2b ). Type 1 cells did not exhibit any voltage-sensitive conductances. Other cells exhibited progressive stages of maturation, from a single broad AP (Type 2), to a full overshooting AP (Type 3), to multiple APs (Type 4). We found that Activin-treated cells could fire APs, and that these neurons fell mainly into Type 2–4 neuronal types ( Fig. 2c ). These results indicate that Activin-treated telencephalic neural precursors can develop into functionally mature neurons. 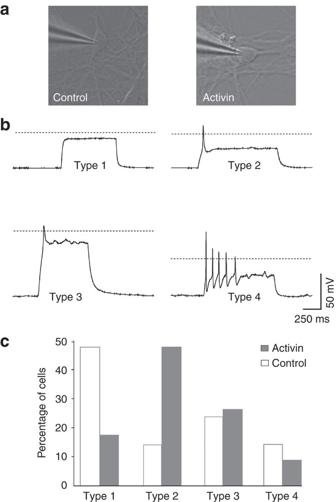Figure 2: Electrophysiological activity of Activin-generated neurons. (a) Representative differential interference contrast images of whole-cell recordings of control and Activin-treated neurons. (b) Representative examples of the four different types of responses of neurons to depolarizing pulses. (c) Activin-treated cells preferentially show an ability to fire APs (82%;n=23), compared with controls (52%;n=21). ESCs were differentiated for 5 days as a monolayer, then replated into poly-D-lysine/laminin-coated dishes and cultured in NBB27 media (controls) or NBB27+10 ng ml−1Activin. Scale bar=10 μm. Figure 2: Electrophysiological activity of Activin-generated neurons. ( a ) Representative differential interference contrast images of whole-cell recordings of control and Activin-treated neurons. ( b ) Representative examples of the four different types of responses of neurons to depolarizing pulses. ( c ) Activin-treated cells preferentially show an ability to fire APs (82%; n =23), compared with controls (52%; n =21). ESCs were differentiated for 5 days as a monolayer, then replated into poly- D -lysine/laminin-coated dishes and cultured in NBB27 media (controls) or NBB27+10 ng ml −1 Activin. Scale bar=10 μm. Full size image The Shh pathway is inhibited by Activin Shh has been widely described as a mitogenic factor for neuronal precursors, both in vivo and in vitro [1] , and is required to maintain stem cell-derived neural precursors during rosette growth [18] . We therefore analysed if Shh signalling has a similar role in telencephalic neural precursors. We found that treatment of these cells with Shh increased the proportion of neural precursors and decreased the proportion of neurons ( Fig. 3a ). In contrast to this, treatment with cyclopamine (a specific Shh pathway inhibitor) lead to the opposite effect ( Fig. 3a ). To test if Shh signalling was affecting the proliferation of neural precursors, analysis of double BrdU + /Nestin + cells was done after a 6-h BrdU pulse. We found that in the presence of exogenous Shh, there was a significant increase in the proportion of double-positive cells and Shh inhibition with cyclopamine led to a dramatic decrease in the number of neuronal precursors that incorporated BrdU ( Fig. 3a ). These results indicate that Shh is mitogenic to telencephalic neural precursors. 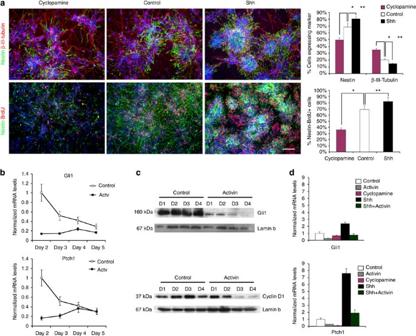Figure 3: Activin antagonizes the mitogenic effects of Shh. (a) Immunostaining (left panels) and quantifications (right panel) indicating that Shh promotes and cyclopamine inhibits proliferation in neural precursors (Nestin+/β-III-tubulin+cells in cyclopamine 49±4.3/35.1±1.8%, Shh 80.3±3.2/14.8±0.7% and control cultures 68.4±7.2/20.1±2.8%;n=3, mean±s.e.m.). (b) Relative expression levels ofGli1andPtch1during the first 5 days of Activin or control treatment. (c) Immunoblot analysis of Gli1 and Cyclin D1 levels during the first 4 days of Activin or control treatment illustrating how Activin represses the expression of these proteins. (d) Normalized mRNA levels ofGli1andPtch1after 24 h exposure to the indicated conditions illustrating how Shh induces the expression of these genes and Activin inhibits their expression (n=3, mean±s.e.m. Student'st-test. *P<0.005 and **P<0.05). ESCs were differentiated for 5 days as a monolayer, then replated into poly-D-lysine/laminin-coated dishes and cultured in NBB27 media (controls), NBB27+10 ng ml−1Activin, NBB27+100 ng ml−1Shh, NBB27+10 μm cyclopamine or NBB27 + 10 ng ml−1Activin + 100 ng ml−1Shh. Scale bar=50 μm. Figure 3: Activin antagonizes the mitogenic effects of Shh. ( a ) Immunostaining (left panels) and quantifications (right panel) indicating that Shh promotes and cyclopamine inhibits proliferation in neural precursors (Nestin + /β-III-tubulin + cells in cyclopamine 49±4.3/35.1±1.8%, Shh 80.3±3.2/14.8±0.7% and control cultures 68.4±7.2/20.1±2.8%; n =3, mean±s.e.m.). ( b ) Relative expression levels of Gli1 and Ptch1 during the first 5 days of Activin or control treatment. ( c ) Immunoblot analysis of Gli1 and Cyclin D1 levels during the first 4 days of Activin or control treatment illustrating how Activin represses the expression of these proteins. ( d ) Normalized mRNA levels of Gli1 and Ptch1 after 24 h exposure to the indicated conditions illustrating how Shh induces the expression of these genes and Activin inhibits their expression ( n =3, mean±s.e.m. Student's t -test. * P <0.005 and ** P <0.05). ESCs were differentiated for 5 days as a monolayer, then replated into poly- D -lysine/laminin-coated dishes and cultured in NBB27 media (controls), NBB27+10 ng ml −1 Activin, NBB27+100 ng ml −1 Shh, NBB27+10 μm cyclopamine or NBB27 + 10 ng ml −1 Activin + 100 ng ml −1 Shh. Scale bar=50 μm. Full size image To investigate the mechanism of how Activin promotes telencephalic neuronal precursor differentiation, we analysed if Shh signalling was affected in Activin-treated neural precursors. Gli1 and Ptch1 are two targets of the Shh signalling pathway [1] . The expression of both these genes is high in control cultures at day 2, correlating with the rapid proliferation of the cells at this stage, and then decreases as terminal differentiation increases in these cultures ( Fig. 3b ). In contrast to this, Activin-treated cells show very low levels of expression of these genes throughout the whole-culture period ( Fig. 3b,c ), suggesting that Activin is inhibiting their expression. Cyclin D1 has also been shown to be a target of Shh signalling in neural precursor cells [19] . We observed the levels of Cyclin D1 protein expression to be high in control cells throughout the culture period. However, in Activin-treated cells Cyclin D1 protein levels were dramatically reduced ( Fig. 3c ), further supporting the concept that Activin is inhibiting Shh signalling. To further test the ability of Activin to repress the Shh pathway, day 2 control cultures were treated with Activin, Shh, cyclopamine or with Shh plus Activin for 24 h. We observed that the expression of Gli1 and Ptch1 was significantly reduced by Activin under these conditions, and that this reduction was comparable to that achieved by cyclopamine treatment ( Fig. 3d ). Therefore, our results suggest that in telencephalic neural precursors Activin is initiating differentiation by directly blocking the mitogenic effects of Shh signalling. Inhibition of Shh signalling by Activin requires Gli3 Gli3 is the main repressor of the Shh pathway during telencephalic development [8] . The Activin signal transducer Smad2 can bind to Gli3R and inhibit its activity; however, upon TGFβ stimulation this interaction is interrupted and Gli3R is released to inhibit Shh signalling [20] . This raises the possibility that Activin may inhibit the Shh pathway via Gli3. To test this, we used ESCs that carry a null mutation in Gli3 [21] . Gli3 −/− neuronal cultures showed enhanced proliferation and displayed an increase in Nestin-expressing neural precursors when compared with wild-type cells ( Supplementary Fig. S3a,b ). We found that in contrast to what occurs with wild-type cells, Activin was unable to induce differentiation in Gli3 −/− neural precursor cultures ( Supplementary Fig. S3a,b ). The low efficiency of neuronal differentiation observed in Gli3 −/− cells even after Activin treatment is likely to be due to a hyperactivation of the Shh pathway as we observe an upregulation of the transcription of the Shh targets Gli1 , Ptch1 and Nkx2.1 in Gli3 −/− cells that is unaffected by Activin treatment ( Supplementary Fig. S3c,d ). Together, these results indicate that Activin requires Gli3 to inhibit the Shh pathway. To further address the interaction between Activin and the Shh pathway, we blocked Shh signalling in Gli3 −/− neuronal cultures using cyclopamine. Interestingly, we found that while cyclopamine increased differentiation in these cells, it induced a significantly lower proportion of neurons than Activin did in control cells ( Fig. 4a versus Fig. 1a ). Therefore, Activin must have other pro-differentiation roles in addition to suppressing Shh signalling. In support of this, the combination of cyclopamine and Activin treatment led to differentiation levels of Gli3 −/− neural precursors that were similar to those observed in Activin-treated control cells ( Fig. 4a versus Fig. 1a ). This indicates three inferences: (1) that Activin needs to suppress Shh signalling to induce differentiation; (2) that Activin inhibits Shh signalling via Gli3; and (3) that, in addition to inhibiting the Shh pathway, Activin must be performing other roles. 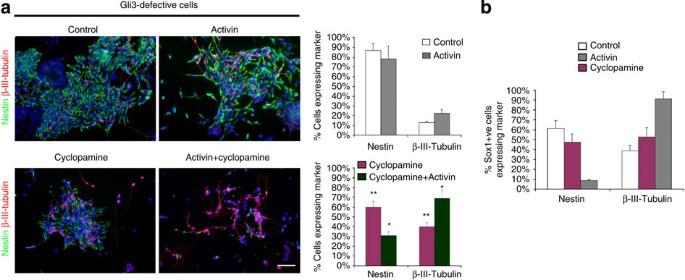Figure 4: Gli3-defective cells do not differentiate in response to Activin. (a) Immunofluorescent images (left panels) and quantification (right panels) of Nestin+and β-III-tubulin+cells in Gli3-deficient neural precursors after 5 days of Activin or control treatment. In these cells, Activin can only induce differentiation once Shh signalling is repressed (Nestin+/β-III-tubulin+cells were 86.7±7/13.2±1.5% in control treated, 78.3±5.2/21.7±4.2% in Activin treated, 60±6/40±4% in cyclopamine treated and 31.5±3.45/70.6±13% in cyclopamine+Activin treated Gli3−/−ESCs). (b) Analysis of Sox1+-sorted wild-type cells after control, cyclopamine or Activin treatment. A higher proportion of these cells differentiate in response to Activin than to cyclopamine (Nestin+/β-III-tubulin+cells in controls 61.3±6.3/38.7±4.64%; in cyclopamine treated 47.2±4.2/52.8±4.2% and in Activin treated 8.7±1.7/91.3±1.7%). For all experimentsn=3, average±s.e.m.; Student'st-test compared with control treatment. *P<0.005 and **P<0.05. ESCs were differentiated for 5 days as a monolayer, then replated into poly-D-lysine/laminin-coated dishes and cultured in NBB27 media (controls), NBB27+10 ng ml−1Activin, NBB27+10 μm cyclopamine or NBB27+10 μm cyclopamine+10 ng ml−1Activin. For (b), Sox+cells were sorted at day 5 of monolayer differentiation and replated as above. Scale bar=25 μm. Figure 4: Gli3-defective cells do not differentiate in response to Activin. ( a ) Immunofluorescent images (left panels) and quantification (right panels) of Nestin + and β-III-tubulin + cells in Gli3-deficient neural precursors after 5 days of Activin or control treatment. In these cells, Activin can only induce differentiation once Shh signalling is repressed (Nestin + /β-III-tubulin + cells were 86.7±7/13.2±1.5% in control treated, 78.3±5.2/21.7±4.2% in Activin treated, 60±6/40±4% in cyclopamine treated and 31.5±3.45/70.6±13% in cyclopamine+Activin treated Gli3 −/− ESCs). ( b ) Analysis of Sox1 + -sorted wild-type cells after control, cyclopamine or Activin treatment. A higher proportion of these cells differentiate in response to Activin than to cyclopamine (Nestin + /β-III-tubulin + cells in controls 61.3±6.3/38.7±4.64%; in cyclopamine treated 47.2±4.2/52.8±4.2% and in Activin treated 8.7±1.7/91.3±1.7%). For all experiments n =3, average±s.e.m. ; Student's t -test compared with control treatment. * P <0.005 and ** P <0.05. ESCs were differentiated for 5 days as a monolayer, then replated into poly- D -lysine/laminin-coated dishes and cultured in NBB27 media (controls), NBB27+10 ng ml −1 Activin, NBB27+10 μm cyclopamine or NBB27+10 μm cyclopamine+10 ng ml −1 Activin. For ( b ), Sox + cells were sorted at day 5 of monolayer differentiation and replated as above. Scale bar=25 μm. Full size image To confirm this third hypothesis, we directly compared the effects of Activin and Shh inhibition on telencephalic neural precursor cells. When Sox1–GFP cells were sorted and treated with Activin or cyclopamine, we observed that while cyclopamine produced only a relatively minor change in the proportion of neural precursors and neurons in the cultures, Activin induced high levels of differentiation ( Fig. 4b ). Therefore, inhibition of Shh alone could not explain the full range of differentiation effects displayed by Activin. Activin enhances the response to RA signalling RA is essential for telencephalic development and acts as a pro-differentiation factor in a wide variety of neuronal settings [2] . Conversion of retinaldehyde to RA is regulated by the Aldh1a subfamily of proteins, and during telencephalic specification the transcription of these factors is controlled by the Activin signal transducer Foxh1 [22] . Therefore, we tested if the regulation of RA signalling could be an additional mechanism that explains Activin's pro-differentiation effect. We first analysed the efficiency with which Activin could induce the differentiation of neural precursors in the absence of exogenous vitamin A (VitA), the RA precursor. For this, we carried out neural differentiation assays using VitA/retinol-deficient B27. We found that while Activin could efficiently induce differentiation when assays were carried out in the presence of VitA, it was unable to induce differentiation in its absence ( Fig. 5a ). In contrast, the differentiation induced by inhibiting Shh signalling with cyclopamine was not significantly affected by the absence of exogenous VitA ( Fig. 5a ). To test which receptors were mediating the RA response, we inhibited RAR and RXR signalling with small-molecule antagonists. When this was done, we observed that while inhibition of the RAR receptors significantly reduced the amount of differentiation induced by Activin, blocking the RXR receptors did not ( Fig. 5b ). Together, these data argue that enhancing RA signalling is one way by which Activin induces differentiation and that this role must be independent of the inhibition of Shh signalling. 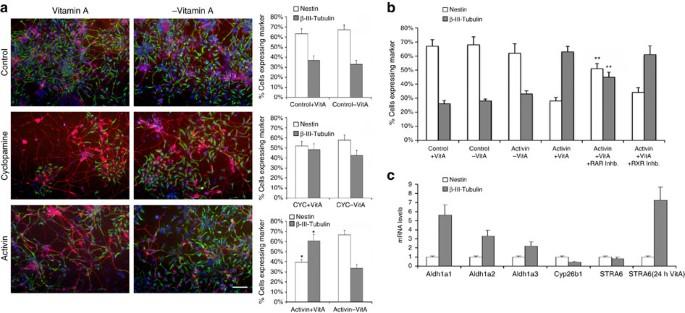Figure 5: Activin enhances RA signalling. (a) Analysis of Nestin and β-III-tubulin immunostaining after 4 days of treatment with control conditions, Activin or cyclopamine in the presence or absence of exogenous RA (VitA). Charts on the right show the quantification for each treatment and illustrate that while cyclopamine can induce differentiation in the absence of exogenous VitA, Activin cannot (Nestin+/β-III-tubulin+cells, +VitA: control 63±3.7/36±4.2%; Activin 39±3.5/60±8%; cyclopamine 51.8±4.43/48.12±4% treated cells. Minus VitA: control 67±5.2/31±2%; Activin 66.4±4.8/33±7%; and cyclopamine-treated cells 57.5±4.1/42±4.8%). (b) Quantification of the proportion of neural precursors and neurons indicates that inhibition of RAR but not RXR blocks the neural differentiation induced by Activin. Nestin+/β-III-tubulin+cells: +VitA=67±4.69/26±2.34%; −VitA=68±5.73/28±1.39%; −VitA+Actv=62±6.71/33±2.2%; +VitA+Actv=28±2.54/63±3.9%; +VitA+Actv+RAR inhibitor=51±3.57/45±3.51% (**P<0.005 for the comparison between +VitA+Act and +VitA+Act+RAR inhibitor); +VitA+Actv+RXR inhibitor=34±3.43/61±6.21%. (c) Quantitative reverse transcriptase PCR analysis indicating how the expression of theAldh1family of genes are promoted by Activin signalling whileCyp26b1is repressed. The RA target geneStra6is only upregulated by Activin in the presence of VitA, suggesting that Activin enhances the response to RA rather than increases RA signallingper se. (c)n=3, average±s.e.m. Student'st-test compared with control treatment. *P<0.05 and **P<0.005. For (a,b), ESCs were differentiated for 5 days as a monolayer, then replated into poly-D-lysine/laminin-coated dishes and cultured in NBB27 media (controls), NBB27+10 ng ml−1Activin, NBB27+10 μm cyclopamine, NBB27+10 μm RXR inhibitor, NBB27+10 μm RXR inhibitor+10 ng ml−1Activin, NBB27+10 μm RAR inhibitor or NBB27+10 μm RAR inhibitor+10 ng ml−1Activin. The NBB27 media were either VitA deficient or supplemented with VitA for these experiments. For (c), ESCs were differentiated for 7 days as a monolayer in NBN2 and B27 minus VitA, then replated into poly-D-lysine/laminin-coated dishes and cultured for 4 days in NBB27 (VitA deficient) media (controls), or NBB27 (VitA deficient)+10 ng ml−1Activin. STRA6 expression was analysed in these samples after being switched to NBB27 (+VitA) media and cultured for a further 24 h. Scale bar=50 μm. Inhb., inhibition. Figure 5: Activin enhances RA signalling. ( a ) Analysis of Nestin and β-III-tubulin immunostaining after 4 days of treatment with control conditions, Activin or cyclopamine in the presence or absence of exogenous RA (VitA). Charts on the right show the quantification for each treatment and illustrate that while cyclopamine can induce differentiation in the absence of exogenous VitA, Activin cannot (Nestin + /β-III-tubulin + cells, +VitA: control 63±3.7/36±4.2%; Activin 39±3.5/60±8%; cyclopamine 51.8±4.43/48.12±4% treated cells. Minus VitA: control 67±5.2/31±2%; Activin 66.4±4.8/33±7%; and cyclopamine-treated cells 57.5±4.1/42±4.8%). ( b ) Quantification of the proportion of neural precursors and neurons indicates that inhibition of RAR but not RXR blocks the neural differentiation induced by Activin. Nestin + /β-III-tubulin + cells: +VitA=67±4.69/26±2.34%; −VitA=68±5.73/28±1.39%; −VitA+Actv=62±6.71/33±2.2%; +VitA+Actv=28±2.54/63±3.9%; +VitA+Actv+RAR inhibitor=51±3.57/45±3.51% (** P <0.005 for the comparison between +VitA+Act and +VitA+Act+RAR inhibitor); +VitA+Actv+RXR inhibitor=34±3.43/61±6.21%. ( c ) Quantitative reverse transcriptase PCR analysis indicating how the expression of the Aldh1 family of genes are promoted by Activin signalling while Cyp26b1 is repressed. The RA target gene Stra6 is only upregulated by Activin in the presence of VitA, suggesting that Activin enhances the response to RA rather than increases RA signalling per se . ( c ) n =3, average±s.e.m. Student's t -test compared with control treatment. * P <0.05 and ** P <0.005. For ( a,b ), ESCs were differentiated for 5 days as a monolayer, then replated into poly- D -lysine/laminin-coated dishes and cultured in NBB27 media (controls), NBB27+10 ng ml −1 Activin, NBB27+10 μm cyclopamine, NBB27+10 μm RXR inhibitor, NBB27+10 μm RXR inhibitor+10 ng ml −1 Activin, NBB27+10 μm RAR inhibitor or NBB27+10 μm RAR inhibitor+10 ng ml −1 Activin. The NBB27 media were either VitA deficient or supplemented with VitA for these experiments. For ( c ), ESCs were differentiated for 7 days as a monolayer in NBN2 and B27 minus VitA, then replated into poly- D -lysine/laminin-coated dishes and cultured for 4 days in NBB27 (VitA deficient) media (controls), or NBB27 (VitA deficient)+10 ng ml −1 Activin. STRA6 expression was analysed in these samples after being switched to NBB27 (+VitA) media and cultured for a further 24 h. Scale bar=50 μm. Inhb., inhibition. Full size image We next analysed how Activin modulates RA signalling and for this we asked if it was regulating the expression of components of the RA pathway. We observed that Activin increased the expression of the Foxh1 targets Aldh1a1-3 ( Fig. 5c ) and inhibited the expression of the RA degrading enzyme Cyp26b1 in neural precursors cultured in the absence of VitA ( Fig. 5b ). In contrast to this, Activin did not affect the expression of the RA responsive gene Stra6 ( Fig. 5b ), indicating that although Activin was controlling the expression of key components of the RA pathway, it was not regulating the expression of genes downstream of RA signalling. To test the physiological importance of this regulation, we asked if the increase in expression of RA pathway components by Activin enhanced the potential of telencephalic neural precursors to respond to RA. For this, we cultured these precursors in the absence of VitA, with or without Activin for 4 days, then treated the cells with VitA for 24 h and analysed Stra6 expression. We observed that cells that had been pre-treated with Activin showed 7 times higher Stra6 expression compared with untreated cells ( Fig. 5b ), indicating that Activin sensitizes telencephalic neural precursors to RA signalling by increasing the ability of these cells to metabolize VitA and decreasing the degradation of RA. Our data suggest that the neurogenic effects of Activin are due to the coordinated inhibition of the Shh pathway and the enhancement of the RA response. For this reason, telencephalic neuronal precursors were treated with cyclopamine and with increased concentrations of RA to see if this would mimic the effects of Activin. We observed that although RA did not induce differentiation, the combination of cyclopamine and 10 μm RA significantly increased the differentiation of neuronal precursors when compared with cyclopamine-treated cells ( Supplementary Fig. S4 ). This synergistic effect suggests that the pro-differentiation role of Activin is mainly due to a repression of Shh pathway and to an enhancement of the response to RA signalling. Induction of CGE identity by Activin To establish if Activin confers positional identity to telencephalic neuronal precursors, we analysed the expression of characteristic patterning markers of the telencephalon. At 12.5 d.p.c., roughly the equivalent stage of the endpoint of our neuronal differentiation assays, the telencephalon is divided into the cortical plate, found dorsally, and the ganglionic eminences, located ventrally. The ganglionic eminences are in turn subdivided into the MGE found in a ventral location, the LGE and the CGE. These regions can also be distinguished molecularly, with Pax6 being expressed in the pallium, Nkx2.1 in the MGE and Gsx2 showing higher levels of expression in the LGE and CGE. Specification of the MGE requires Shh signaling, and Nkx2.1 has been shown to be a Shh target [23] , [24] , [25] . In agreement with the role of Activin in suppressing Shh signalling, we found that Activin caused a fivefold repression in Nkx2.1 expression in telencephalic neuronal cultures, an inhibition similar to that seen with cyclopamine treatment ( Fig. 6a ). A similar downregulation was observed in the expression of Lhx6 , a marker of postmitotic migrating MGE-derived neurons [26] , [27] , after Activin treatment ( Fig. 6a ), indicating that unlike control cultures, Activin treatment was not leading to the acquisition of an MGE fate. We next examined the expression of Pax6 , whose expression is promoted by cyclopamine and suppressed by Shh in ESC-derived telencephalic neural cultures [14] , [28] and found that Activin had little effect on its expression ( Fig. 6a ). In contrast to this and unlike what occurs in control cultures, or after Shh or cyclopamine treatment, we observed that Activin caused a 13-fold increase in the mRNA expression of Gsx2 and a 7-fold increase in the proportion of Gsx2-expressing cells ( Fig. 6a–b ). This suggests that Activin is inducing telencephalic precursors to adopt an LGE/CGE fate. 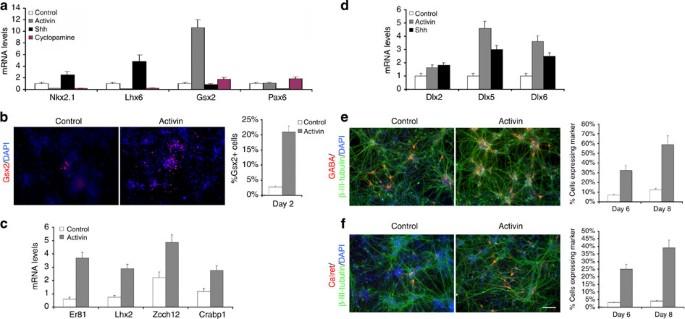Figure 6: Activin provides telencephalic neuronal precursors with a CGE identity. (a) Quantitative reverse transcriptase PCR analysis of telencephalic gene expression indicates that Activin promotesGsx2and inhibitsNkx2.1andLhx6expression. (b) Immunofluorescent analysis (left panel) and quantification (right panel) of Gsx2+cells indicates that Activin induces this cell type (control 2.8±0.3% and Activin treated 21±1.9%). (c) Normalized mRNA levels of CGE genes and (d)Dlxgene expression indicating that Activin induces the expression of these genes. (e) Immunofluorescent images (left panels) and quantification (right panel) of β-III-tubulin/GABA double-positive cells (control day 6: 5.84±0.5%; control day 8: 12.51±1.18%; Activin day 6: 31.29±1.18%; Activin day 8: 58.93±−7.2%) and (f) β-III-tubulin/calretinin double-positive cells (control day 6: 3.3±0.12%; control day 8: 4.2±0.4%; Activin day 6: 25±6.2%; Activin day 8: 38.72±4.3%) illustrating how Activin promotes the development of GABAergic calretinin-positive interneurons. For all experimentsn=3, mean±s.e.m. ESCs were differentiated for 5 days as a monolayer, then replated into poly-D-lysine/laminin-coated dishes and cultured in NBB27 media (controls) or NBB27+10 ng ml−1Activin for 3 days (a), 2 days (b), 4 days (c,d) or 6–8 days (e,f). BDNF (10 ng ml−1) was added from day 7 after re-plating. Scale bar=50 μm. Figure 6: Activin provides telencephalic neuronal precursors with a CGE identity. ( a ) Quantitative reverse transcriptase PCR analysis of telencephalic gene expression indicates that Activin promotes Gsx2 and inhibits Nkx2.1 and Lhx6 expression. ( b ) Immunofluorescent analysis (left panel) and quantification (right panel) of Gsx2 + cells indicates that Activin induces this cell type (control 2.8±0.3% and Activin treated 21±1.9%). ( c ) Normalized mRNA levels of CGE genes and ( d ) Dlx gene expression indicating that Activin induces the expression of these genes. ( e ) Immunofluorescent images (left panels) and quantification (right panel) of β-III-tubulin/GABA double-positive cells (control day 6: 5.84±0.5%; control day 8: 12.51±1.18%; Activin day 6: 31.29±1.18%; Activin day 8: 58.93±−7.2%) and ( f ) β-III-tubulin/calretinin double-positive cells (control day 6: 3.3±0.12%; control day 8: 4.2±0.4%; Activin day 6: 25±6.2%; Activin day 8: 38.72±4.3%) illustrating how Activin promotes the development of GABAergic calretinin-positive interneurons. For all experiments n =3, mean±s.e.m. ESCs were differentiated for 5 days as a monolayer, then replated into poly- D -lysine/laminin-coated dishes and cultured in NBB27 media (controls) or NBB27+10 ng ml −1 Activin for 3 days ( a ), 2 days ( b ), 4 days ( c,d ) or 6–8 days ( e,f ). BDNF (10 ng ml −1 ) was added from day 7 after re-plating. Scale bar=50 μm. Full size image The most ventral part of the LGE is characterized by low expression of Gsx2 and the absence of Er81 expression and later by increased Islet1 expression. The most dorsal part of the LGE expresses Gsx2 and Er81 . The CGE has been recently described as a prolongation of the LGE region and of part of the MGE [9] , [29] , [30] . We observed that Activin-treated cells did not show any increase in Islet1 expression (data not shown), but did show a fivefold increase in Er81 expression compared with controls ( Fig. 6c ), suggesting a dorsal LGE or CGE fate. To better discriminate between LGE and CGE, we analysed the expression of genes that has been previously found enriched in CGE when compared with LGE [31] , [32] , [33] . We found the expression of Lhx2 , Zcchc12 and Crabp1 also to be upregulated in Activin-treated cells ( Fig. 6c ), and that the proportion of neural progenitors and neurons expressing CoupTFII (a gene expressed preferentially in the CGE [9] , [32] ) increased upon Activin treatment ( Supplementary Fig. S5a ), supporting that the telencephalic progenitors in these cultures were acquiring a CGE identity. The CGE produces calretinin-positive GABAergic interneurons that will migrate to the cortex [27] , [29] , [34] , [35] , [36] . The homeobox genes Dlx2 , Dlx5 and Dlx6 are expressed in all developing and mature cortical interneurons throughout the subpallial domain as well as in a number of other non-cortical neuronal cell types [37] , [38] . We observed that Activin treatment increased the levels of expression of all these genes ( Fig. 6d ) and 52±5% of Activin-treated cells were Dlx2 expressing ( Supplementary Fig. S5b ). Activin treatment also resulted in a fivefold increase in the proportion of GABA + /ßβ-III-tubulin + neurons ( Fig. 6e ) and a dramatic enrichment in calretinin + /ßβ-III-tubulin + cells ( Fig. 6f ). To enhance the maturation of these interneurons, Brain Derived Neurotrophic Factor (BDNF) was added from day 7 to 12 of differentiation. This led to 76.34±6.8% of calretinin-expressing neurons also expressing GABA ( Supplementary Fig. S5c ) and 67.6±6.5% expressing GAD67 (data not shown). In contrast to this, we observed that only 0.001% of Activin-treated neurons expressed other interneuron markers, such as somatostatin (data not shown). Of the calretinin-positive neurons, <5% expressed tyrosine hydroxylase, ruling out they could be olfactory bulb interneurons of the glomerular layer ( Supplementary Fig. S5c and S5c' ), and 95.7±5% of them expressed the CGE marker COUP-TFII ( Supplementary Fig. S5d ). Interestingly, we also observed that Activin treatment led to an enrichment in the proportion of Reelin-expressing cells, another type of interneurons derived from the CGE (control: 6±0.5% and in Activin-treated cells: 14.38%±1.2; Supplementary Fig. S5e,f ). The observation that only a small proportion of calretinin-positive neurons also expressed Reelin (16±1.44%; Supplementary Fig. S5e,f ) indicates that these cells are not Cajal Retzious neurons. Together, these observations strongly suggest that Activin is promoting CGE identity and the formation of cortical calretinin interneurons derived from this subregion of the forebrain. To address if the neurons we generate by Activin treatment can survive and integrate in vivo , we injected these neurons into the somatosensory cortex of adult mice. We observed that telencephalic neural precursors derived from Activin-treated, GFP-labelled ESCs could be observed 1 month after transplantation, predominantly adjacent to the site of injection ( Supplementary Fig. S6a ). Interestingly, those cells that were found away from the site of injection expressed calretinin, were vertically oriented and bipolar ( Supplementary Fig. S6b ), supporting our conclusions that they are likely calretinin interneurons. Remarkably, these neurons formed both dendrites and dendritic spines, suggesting that they are mature and physiologically active neurons ( Supplementary Fig. S6c ). Together, these data suggest that the calretinin neurons generated by Activin treatment of ESC-derived telencephalic neuronal precursors are able to integrate in vivo and are physiologically active. A conserved role for Activin in human pluripotent stem cells To determine if the roles of Activin in inducing neuronal precursor differentiation, providing a CGE fate and calretinin interneuron identity are conserved in humans, we analysed the effect that Activin treatment has on telencephalic neural precursors derived from two independent lines of human ESCs (H1 and H7) or two independent lines of human-induced pluripotent stem cells (iPSCs) (2F8 and 4FHuang). Human embryonic stem cells (hESCs) were differentiated along a neural lineage as previously described [39] . Using this protocol, in H7 cells at day 17, the expression of pluripotency markers is extinguished and the majority of the cells become telencephalic neural precursors expressing SOX1 and PAX6 ( Supplementary Fig. S7a,c ). At day 19, cells were replated on poly- D -lysine- and laminin-coated dishes and treated with Activin for 6 days. In H1 and the IPSCs, differentiation occurred more rapidly and therefore Activin was added at day 9 for 6 days ( Supplementary Fig. S7a ). We first analysed the pro-differentiation capacity of Activin in H7 hESCs and found that similar to what occurred in mouse ESCs, Activin treatment reduced the proportion of Nestin-positive neural precursors and increased the proportion of âβ-III-tubulin neurons ( Fig. 7a,b ). Similar results were obtained with the H1 and IPSC lines (data not shown). This indicated that Activin also induces neuronal differentiation of human pluripotent stem cells. We next tested if Activin could inhibit the targets of Shh signalling as well as if it is required for RA signalling during the differentiation of neural precursors derived from human ESCs. We found that, while a 6-day Activin treatment resulted in a moderate inhibition of the Shh targets PTCH1 and GLI1 in hESC-derived neural progenitors, Activin clearly suppressed PTCH1 and GLI1 induction by exogenous Shh ( Supplementary Fig. S8a ). In these cells, we also observed an upregulation of Aldh1a1 and a repression of Cyp26b1 ( Supplementary Fig. S8b ), suggesting that RA signalling was enhanced. To further test if RA signalling is required for Activin to induce neuronal differentiation in neural precursors derived from hESCs, we either performed the differentiations in the absence of exogenous RA, in the presence of an RAR inhibitor or in the presence of an RXR inhibitor. We observed that as with mouse ESCs, the ability of Activin to induce differentiation was compromised in the absence of RA or by inhibition of the RAR receptors, but that blocking the RXR receptors had little effect on the ability of Activin to induce differentiation ( Supplementary Fig. S8c,d ). Interestingly, we observed that the combination of both RAR and RXR inhibitors led to the death of the telencephalic neural precursors derived from mESCs and hESCs (data not shown). This contrasts with what is seen with precursors of the spinal cord derived from hESCs [40] , suggesting that neural precursors with different regional identity are differentially sensitive to the pan-inhibition of RA receptor signalling. In conclusion, we observe that both in mESCs and hESCs Activin requires RA signalling via the RAR receptors to promote differentiation. 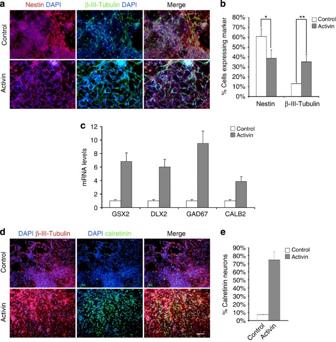Figure 7: The roles of Activin are conserved in hESCs. (a) Immunostaining and (b) quantification indicating that Activin induces the differentiation of neural precursors derived from human ESCs (Nestin+/β-III-tubulin+cells: control 60±7/13±1.6% and Activin-treated cells 38±8/35±7.7%). (c) Quantitative reverse transcriptase PCR analysis of the expression ofGSX2, DLX2, GAD67 and CALB2indicating that Activin promotes the expression of these genes. (d) Immunostaining and (e) quantification of β-III-tubulin/calretinin double-positive cells indicating that Activin promotes the formation of calretinin interneurons from neural precursors derived from human ESCs (control 7.18±0.35%; Activin-treated cells 74.5±4.2%). For all experimentsn=3, mean±s.e.m. Student'st-test compared with control treatment. *P<0.05 and **P<0.005. hESCs were differentiated in N2B27 with 100 ng ml−1noggin, 10 μm SB431542 and 200 nM dorsomorphin for 4 days (H1/IPSCs) or for 5 days (H7), then cultured in N2B27 with 100 ng ml−1noggin and 200 nM dorsomorphin for 3 days (H1/IPSCs) or 4 days (H7) and after a further 2 days, culture in N2B27 alone cells were passaged. At this stage, cells were replated into fibronectin-coated dishes and cultured in N2B27 for a further 2 days (H1/IPSCs) or 10 days (H7) and split again. Cells were then replated into poly-L-lysine/laminin-coated dishes and cultured in N2B27 (controls) or N2B27+10 ng ml−1Activin for 6 days (H1/iPSCs) or 7 days (H7). Scale bar=25 μm (a) and 50 μm (d). Figure 7: The roles of Activin are conserved in hESCs. ( a ) Immunostaining and ( b ) quantification indicating that Activin induces the differentiation of neural precursors derived from human ESCs (Nestin + /β-III-tubulin + cells: control 60±7/13±1.6% and Activin-treated cells 38±8/35±7.7%). ( c ) Quantitative reverse transcriptase PCR analysis of the expression of GSX2, DLX2, GAD67 and CALB2 indicating that Activin promotes the expression of these genes. ( d ) Immunostaining and ( e ) quantification of β-III-tubulin/calretinin double-positive cells indicating that Activin promotes the formation of calretinin interneurons from neural precursors derived from human ESCs (control 7.18±0.35%; Activin-treated cells 74.5±4.2%). For all experiments n =3, mean±s.e.m. Student's t -test compared with control treatment. * P <0.05 and ** P <0.005. hESCs were differentiated in N2B27 with 100 ng ml −1 noggin, 10 μm SB431542 and 200 nM dorsomorphin for 4 days (H1/IPSCs) or for 5 days (H7), then cultured in N2B27 with 100 ng ml −1 noggin and 200 nM dorsomorphin for 3 days (H1/IPSCs) or 4 days (H7) and after a further 2 days, culture in N2B27 alone cells were passaged. At this stage, cells were replated into fibronectin-coated dishes and cultured in N2B27 for a further 2 days (H1/IPSCs) or 10 days (H7) and split again. Cells were then replated into poly- L -lysine/laminin-coated dishes and cultured in N2B27 (controls) or N2B27+10 ng ml −1 Activin for 6 days (H1/iPSCs) or 7 days (H7). Scale bar=25 μm ( a ) and 50 μm ( d ). Full size image When we analysed how Activin affected the patterning of neural precursors derived from hESCs, we found that it induced a sixfold increase in Dlx2 mRNA levels, a sevenfold stimulation of Gsx2 expression, a ninefold increase in the levels of GAD67 and a fourfold increase in calretinin expression ( Fig. 7c ). Double staining for β-III-tubulin/calretinin indicated that 74.5±4.2% of postmitotic neurons were calretinin positive, a tenfold enrichment with respect to controls ( Fig. 7d,e ). Furthermore, the vast majority of these calretinin neurons expressed GABA (94.73±2.07%; Fig. 7e ). These results suggest that, as occurs with mouse cells, Activin can induce a CGE fate and cortical calretinin interneuron identity in neural precursors derived from hESCs. We also observed that Activin had similar roles during the neuronal differentiation of human-iPSCs ( Supplementary Fig. S7d ). Therefore, the roles of Activin in ESC-derived, forebrain-like neural precursors appears to be conserved between the mouse and humans. Cell replacement therapy using ESCs holds great promise for the treatment of many central nervous system diseases and injuries that to date have little or no therapy available, including traumatic injury, neurodegenerative diseases and stroke. ESCs also provide invaluable tools for drug discovery and for furthering our understanding of the development of the nervous system in health and disease. In this paper, using telencephalic neural precursors derived from mouse and human ESCs, we show that Activin controls two key aspects of neurogenesis, the decision of neural precursors to self-renew or differentiate, and their choice of neuronal subtype identity. Differentiation of neuronal precursors into postmitotic neurons requires the careful coordination of signals that inhibit self-renewal with those that implement the programme of terminal differentiation. The self-renewal of neural precursors is controlled by Shh signalling both in vivo and in vitro [1] . ESC-derived neural precursors display endogenous Shh activity [14] and this activity is required to maintain stem cell-derived neural precursors during rosette growth [18] . In this work, we show that the crosstalk between Shh and Activin signalling controls the balance between self-renewal and differentiation of telencephalic neural precursors derived from ESCs. We find that in these cells Shh is a potent mitogenic factor and that Activin induces differentiation by inhibiting Shh signalling in a Gli3-dependent manner and in this way initiates the differentiation process ( Fig. 8 ). 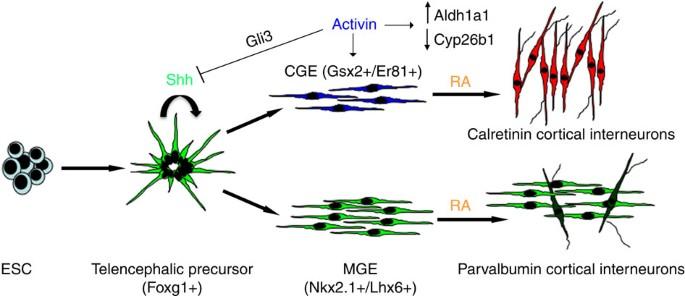Figure 8: Model for how Activin induces the differentiation and CGE fate in telencephalic neuronal precursors. Our work suggests that during the neuronal differentiation of neural precursors Activin has three roles. First Activin inhibits Shh signalling in a Gli3-dependent manner. Second, Activin enhances the response of telencephalic neural precursors to RA by increasing the expression of genes that promote RA signalling, such as Aldh1a1-3, and by repression of those that inhibit it, such as Cyp26b1. We suggest that these changes result in a sensitization of these precursors to VitA, so that when these cells are presented with VitA they can rapidly undergo differentiation. The third role of Activin during the neuronal process is to promote a calretinin interneuron identity in the differentiating neural precursors. Figure 8: Model for how Activin induces the differentiation and CGE fate in telencephalic neuronal precursors. Our work suggests that during the neuronal differentiation of neural precursors Activin has three roles. First Activin inhibits Shh signalling in a Gli3-dependent manner. Second, Activin enhances the response of telencephalic neural precursors to RA by increasing the expression of genes that promote RA signalling, such as Aldh1a1-3, and by repression of those that inhibit it, such as Cyp26b1. We suggest that these changes result in a sensitization of these precursors to VitA, so that when these cells are presented with VitA they can rapidly undergo differentiation. The third role of Activin during the neuronal process is to promote a calretinin interneuron identity in the differentiating neural precursors. Full size image The second way by which Activin induces differentiation is by enhancing the response of telencephalic neural precursors to RA, the pathway that implements neurogenic differentiation [2] ( Fig. 8 ). We find that Activin treatment leads to an increase in the expression of genes that promote RA signalling, such as Aldh1a1-3 , that have already been shown to be direct targets of Activin signalling in the forebrain [22] , and to a repression of those that inhibit it, such as Cyp26b1 . We suggest that these changes result in a sensitization of the telencephalic neural precursors to VitA, so that when these cells are presented with VitA they can rapidly undergo differentiation. By inhibiting the pathway that controls self-renewal and enhancing the response to the pro-neurogenic pathway, Activin ensures that the whole differentiation process of telencephalic neural progenitors is tightly regulated. The fact that in neural precursors derived from hESCs (our work) and in the chick spinal cord [41] , [42] Activin also promotes differentiation suggests that this role may be conserved in a wide variety of neuronal settings. Interestingly, in the chick neural tube the Activin effector Smad3 induces differentiation by activating p27 kip1 expression [42] . However, we observed no change in p27 kip1 expression upon Activin treatment of telencephalic neural precursors derived from ESCs (data not shown), suggesting that the downstream molecular response to Activin signalling varies with the cellular context. In addition to inducing differentiation, we find that Activin provides neural progenitors with neuronal subtype identity ( Fig. 8 ). We show that in telencephalic neural precursors derived both from mouse and human ESCs, Activin regulates the two transcription factors that control interneuron progenitor fate to an LGE/CGE or MGE identity. Activin specifically promotes Gsx2 expression and inhibits Nkx2.1 in these cells, and in this way leads to the acquisition of a CGE fate and calretinin interneuron differentiation. The main growth factor identified so far in determining cortical interneuron fate is Shh. Shh signalling is required for specifying MGE identity and for the formation of somatostatin and parvalbulim interneurons, and loss of Shh signalling leads to increased calretinin interneuron development in vivo [43] . However, although the CGE develops independently of Shh [44] , during ESC differentiation the inhibition of Shh generates glutamatergic neurons and never gives rise to Gsx2 progenitors or calretinin interneurons [14] , [28] . Therefore in addition to inhibiting Shh signalling, Activin must be performing additional roles. Interestingly, the combination of both cyclopamine and RA also fails to increase Gsx2 expression and calretinin interneuron formation in our cultures (data not shown), suggesting that this additional role does not involve the regulation of RA. The finding that treatment of Foxg1 + telencephalic precursors with Fgf15/19 can also generate calretinin interneurons [45] , and that Fgf15 has been shown to be a direct target of Activin signalling in ESCs [46] , suggests that these factors may be directly regulated by Activin during the specification of cortical interneuron fate. It is worth adding that Activin's roles in promoting differentiation and providing cell fate identity does not necessarily imply that these two processes are separable as the regulation of cell fate identity and differentiation are closely interlinked processes. Cortical interneurons are of particular interest for cell transplantation owing to their remarkable migratory capacity in postnatal cortex, their stereotypic differentiation after transplantation and their regulation of cortical activity [10] , [11] , [12] , [13] . They are also involved in a number of neuropsychiatric illnesses, including epilepsy, autism and schizophrenia [11] , [47] . Specifically, it has been suggested that calretinin interneurons may be implicated in epilepsy [11] , [48] . The protocol that we describe in this manuscript represents a method to obtain an enriched source of calretinin interneurons from both mouse and human ESCs. Therefore, our work significantly contributes to the aim of generating the diverse neuronal subtypes required for the safe and successful use of ESCs in regenerative medicine. Cell culture Four mouse ESC lines were used: control E14, Sox1–GFP (46C) and +/+ (that are Gli3 +/+ and therefore a wild-type line derived from the same genetic background as the Gli3 −/− ESCs) and a Gli3-defective line (Xt7). All ESCs were maintained under standard conditions and differentiated as previously described [15] with minor modifications. ESC lines were maintained in 0.1% gelatin-coated flasks with GMEM supplemented with 10% FCS, NEAA, L -Glutamine, Sodium Pyruvate, β-mercaptoethanol (all from Gibco) and LIF (Millipore) and divided 1:8 or 1:10 every 2–3 days. For monolayer neural differentiation, cells were replated at low density (7,500 cells cm −2 ) in NB (neurobasal media, Gibco) supplemented with B27 diluted 1:50 (Gibco), L -Glutamine and β-mercaptoethanol. Media was changed every day and at day 5 of differentiation, cells were split 1:3, replated into Poly- D -lysine/laminin-coated dishes, and maintained in NB media (control cells) or in NB media supplemented with 10 ng ml −1 of Activin (R&D Systems). For the differentiation without RA, N2 was added to the media and cells were maintained on gelatin for 7 days instead of 5, then replated as normally and cultured in the media described. For the RA receptor inhibition, AGN193109 (Santa Cruz) and UVI 3003 (Tocris Bioscience) were used at 10 μm. Cyclopamine (Sigma) was used at 10 μm, Shh (R&D Systems) at 25 ng ml −1 and BDNF (Sigma) at 10 ng ml −1 . Human ESCs H1 and H7 as well as the human IPSC lines 2F8 and 4FHuang were maintained and differentiated as previously described [39] with minor modifications. Human cells were maintained on a feeder layer of Mitomycin C-treated mouse embryonic fibroblasts and passaged weekly by EDTA dissociation. Cells were maintained in KO–DMEM with 15% KO serum replacement (both from Invitrogen) supplemented with 8 ng ml+ of bFGF (Preprotech), NEAA, NaPyr, B-ME and L -glutamine. For neural differentiation, human cells were preplated on gelatin-coated dishes for 60 min to remove contaminating feeder cells and then plated into growth-factor-reduced matrigel-coated plates (BD Biosciences). The basal media used for differentiation was N2B27 with both supplements at a dilution of 1 in 200 (Invitrogen). Neural induction was achieved with 100 ng ml −1 noggin (R&D Systems), 10 μm SB431542 (Sigma) and 200 nM dorsomorphin (Tocris Bioscience). SB431542 was removed from the N2B27 after day 5 and noggin and dorsomorphin were removed after day 9 of differentiation. Pro-neural cells were passaged at day 11 of differentiation using 0.02% EDTA (Sigma) and manual disaggregation. The cells were maintained for a further 9 days before being passaged for a second time. The precursor cells were then plated into fibronectin-coated dishes and cultured with Activin at a concentration of 10 ng ml −1 (R&D Systems). Immunostaining ESCs were fixed with 4% paraformaldehyde for 20 min, and for nuclear antigen detection an additional methanol fixation was used (20 min at −20 o C). Cells were then blocked and permeabilized with 8% BSA+0.2% Tween-20 for 20 min at room temperature, and washed with PBS. Antibodies used were anti-âβ-III-tubulin rabbit polyclonal 1:300 (Abcam), anti-Nestin mouse monoclonal 1:300 (BD transduction), anti-Calretinin rabbit polyclonal 1:400 (Swant) and anti-GABA rabbit polyclonal 1:500 (Sigma), anti-Gsx2 rabbit polyclonal (kindly provided by K. Campbell), anti-Foxg1 rabbit polyclonal 1:400 (Abcam), anti-Dlx2 rabbit polyclonal 1:300 (Millipore), anti-CoupTFII mouse monoclonal 1:300 (R&D Systems), anti-GAD67 mouse monoclonal 1:100 (Millipore) and anti-Reelin mouse monoclonal 1:200 (MBL). Secondary antibodies were Alexa fluor 488 or 568 Donkey anti-rabbit and Donkey anti-mouse (Invitrogen). For Human ESCs, primary antibodies used were Rabbit Tuj1 1:1,000 (Covance), mouse Nestin 1:300 (Neuromics) and rabbit Calretinin 1:400 (Swant), incubated all night at 4 °C in 3% serum. All data were collected from a minimum of three independent differentiation experiments. RNA isolation and RT–PCR Total RNA was extracted using RNeasy (Qiagen). Complementary DNA was synthesized using SuperScript III Reverse Transcriptase (Invitrogen), Random Nonamers (Sigma) and RNAse out (Roche). qPCR was performed with SYBR PCR Master Mix (Qiagen). Standard curves and melting curves were measured for each set of primers to confirm that only one amplicon was generated and β-actin was used as a house keeping gene. The expression levels of mRNA were calculated using the comparative CT method. Primers used are listed in Supplementary Table S1 . Western blotting Cell pellets were resuspended in RIPA buffer and sonicated. Proteins (25–40 μg) were resolved by a 6–12% SDS–PAGE gel and subjected to western blot analysis. Primary antibodies used were anti-Gli1 rabbit polyclonal (Cell Signalling) and anti-Cyclin D1 rabbit polyclonal (Santa Cruz). Electrophysiology Activin-treated and control cells at day 5 were mounted on a recording chamber and bathed with physiological extracellular recording solution (composition in mM, NaCl 147, KCl 3.5, HEPES 10, Glucose 11, MgCl2 2, CaCl2 2, pH=7.4) at room temperature (20–22 °C). Recording sessions from each coverslip were limited to 75 min to ensure maximum membrane integrity and cell viability. Cells were visualized under an upright microscope (Olympus BXWI 51, Japan) equipped with a ×40 objective, an infared filter, differential interference contrast optics and a cathode-cooled diode (CCD) video camera (Hamamatsu Photonics, Germany). Whole-cell current-clamp recordings were performed with an Axopatch 200A amplifier (Axon Instruments, USA) using glass microelectrodes (3–6 MΩ in resistance) filled with an internal solution containing (in mM) 140 K-gluconate, 5 NaCl, 1 MgCl2, 10 HEPES, 1 EGTA, 2 MgATP, 0.5 LiGTP, pH 7.3, osmolarity 280–290 mosmol l −1 . Cells were recorded in current-clamp conditions for a minimum of 1–2 min after breaking into the whole-cell mode to establish their ability to fire APs by delivering depolarizing pulses (10–500 pA, 0.5–2 s duration at around 0.01 Hz). Transplantation in the adult mouse cortex and 2-photon/confocal imaging Mice ( n =2 males, >5-month-old) were given an intraperitoneal injection of an anaesthetic mixture (0.13 mg ketamine/0.01 mg xylazine/g body weight) and a small dose of dexamethasone (i.m., 0.02 ml at 4 mg ml −1 ) and bupivacaine (s.c., 0.125% in saline) immediately before the surgery and transferred to a stereotaxic apparatus (Stoelting). GFP-expressing cells (100,000 cells μl −1 ) were injected through a small craniotomy (4 mm in diameter) over the somatosensory cortex [49] using glass pipettes (tip diameter ~10 μm) filled with 0.5 μl of cell solution. About 10–100 nl volumes were injected using a picospritzer (III, General Valve) and several pressure pulses (20 psi; 15 ms). After a period of 1 month, mice were perfused and brains removed and processed for immunohistochemistry. Immunohistochemistry and 2-photon/confocal imaging Paraformaldehyde-fixed brains were embedded in agarose gel and serial sections cut with a vibrating microtome (Leica). The sections were washed (3×10 min) in permeabilization buffer (0.2% TX100 in PBS) before incubation (>1 h) in blocking buffer (10% NGS and 0.2% TX100 in PBS). Sections were then incubated (overnight at 4 °C) with primary antibodies (rabbit anti-calretinin, 1:500 (Swant)) diluted in blocking buffer. Sections were washed (3×30 min) in PBS + 0.2% TX100 before incubation (>2 h) with secondary antibody (Cy3 conjugated goat anti-rabbit, 1:500). After further washes (3×10 min) in PBS + 0.2% TX100, sections were mounted on glass slides with Vectashield (containing 4',6-diamidino-2-phenylindole) and glass coverslips. Images were obtained using confocal (SP5II, Leica) and 2-Photon (Prairie Technologies) microscopy. How to cite this article: Cambray, S. et al . Activin induces cortical interneuron identity and differentiation in embryonic stem cell-derived telencephalic neural precursors. Nat. Commun. 3:841 doi: 10.1038/ncomms1817 (2012).